Phosphatidylinositol 5-phosphate regulates invasion through binding and activation of Tiam1 PtdIns5P is a lipid messenger acting as a stress-response mediator in the nucleus, and known to maintain cell activation through traffic alterations upon bacterial infection. Here, we show that PtdIns5P regulates actin dynamics and invasion via recruitment and activation of the exchange factor Tiam1 and Rac1. Restricted Rac1 activation results from the binding of Tiam1 DH-PH domains to PtdIns5P. Using an assay that mimics Rac1 membrane anchoring by using Rac1-His and liposomes containing Ni 2+ -NTA modified lipids, we demonstrate that intrinsic Tiam1 DH-PH activity increases when Rac1 is anchored in a PtdIns5P-enriched environment. This pathway appears to be general since it is valid in different pathophysiological models: receptor tyrosine kinase activation, bacterial phosphatase IpgD expression and the invasive NPM-ALK(+) lymphomas. The discovery that PtdIns5P could be a keystone of GTPases and cytoskeleton spatiotemporal regulation opens important research avenues towards unravelling new strategies counteracting cell invasion. Phosphoinositides (PIs) are spatiotemporal organizers of signal transduction, rearrangement of the actin cytoskeleton, intracellular vesicle trafficking and survival [1] , [2] . They have specific localizations within cells that account for recruitment of effectors displaying PI-binding domains such as PH, FYVE, FERM, PHOX and more recently PHD to regulate signalling [3] . Deregulation and mutations in PI-metabolizing enzymes take part in the development of human pathologies including genetic diseases and cancer [4] , [5] . Phosphatidylinositol 5-phosphate (PtdIns5P) metabolism and functions remain poorly understood. It is present at low levels in many cell types, and several physiological and pathophysiological challenges alter PtdIns5P levels, indicating that it is a signalling molecule, in addition to having housekeeping functions [6] , [7] . A large body of studies over the years has focused on nuclear PtdIns5P, identifying it as a stress-induced second messenger that regulates apoptosis by binding the PHD domain of the chromatin-regulator ING2 (refs 8 , 9 ). Cell fractionation demonstrated that while the majority of bulk PtdIns5P is present in the plasma membrane, it is also enriched in intracellular membrane compartments including endosomes, smooth endoplasmic reticulum and the trans-Golgi network [10] , [11] . Our group pioneered studies demonstrating that PtdIns5P was produced upon bacterial infection of HeLa cells by the human pathogens Shigella flexneri and Salmonella typhimurium [12] , [13] . S. flexneri ’s virulence factor, IpgD, is a potent 4-phosphatase that converts PtdIns(4,5)P 2 into PtdIns5P and contributes to dramatic F-actin remodelling, facilitating bacterial entry and inducing alteration of trafficking through PtdIns5P accumulation on early endosomes to maintain host cell activation [10] , [13] , [14] . Additional studies in different models confirmed that PtdIns5P impacts actin reorganization. PtdIns5P produced by the PI 5-kinase PIKfyve was implicated in insulin-induced F-actin breakdown, thereby regulating trafficking of vesicles containing the GLUT4 glucose transporter from intracellular membranes pools to the plasma membrane [15] , [16] , [17] . In line with these observations, recent studies have identified PtdIns5P as the central molecule regulating cell migration in response to FGF-1 in fibroblasts and in border cells during Drosophila embryogenesis, where its production is locally regulated at the endosomal level by the interplay of PIKfyve and the PI 3-phosphatase MTMR3 (ref. 15 ). However, the precise molecular mechanisms linking PtdIns5P to actin dynamics and migration are still unknown. Our previous work on anaplastic lymphomas expressing the tyrosine kinase oncogene NPM-ALK demonstrated that the oncogene activated PIKfyve to produce PtdIns5P. Moreover, invasiveness of NPM-ALK(+) cells was regulated not only by PIKfyve but also by the Rac1 GTPase [18] , [19] , [20] , [21] . Knowing the importance of Rho GTPases as molecular switches regulating a wide array of cellular processes, such as cytoskeleton remodelling, membrane dynamics and migration in response to PIs, they represent ideal candidates to link PtdIns5P to the aforementioned cellular responses [22] , [23] . With those observations in mind, we sought to investigate whether PtdIns5P could activate Rho GTPases signalling and address the functionality of such activation using various models. Three complementary models were used to evaluate the general nature of the mechanism. We first studied FGF-1 stimulation of RPE-1 cells; second, we used the bacterial phosphatase IpgD to produce PtdIns5P in MEFs; and third, we analysed NPM-ALK(+) anaplastic lymphomas. We find that PtdIns5P elevation is responsible for Rac1 activation in all three models and identify the guanine nucleotide exchange factor (GEF) Tiam1 (T-cell lymphoma invasion and metastasis 1) as being activated by PtdIns5P and required for Rac1 activation. We demonstrate that the C-terminal regulatory PH domain (PHc) of Tiam1 binds specifically to PtdIns5P, leading to recruitment of active Tiam1/Rac1 to early endosomes and dorsal ruffles. This is mandatory for robust change in actin and membrane dynamics upon PtdIns5P elevation. Interestingly, elevated levels of PtdIns5P induce invasion in pathophysiological contexts, being even sufficient to trigger invasive capabilities in cells that are otherwise not able to migrate in 3D. These observations broaden the understanding of PtdIns5P by suggesting that it can integrate several upstream signals to coordinate trafficking as well as actin and membrane dynamics to regulate invasion. PtdIns5P induces Rac1 and Cdc42 activation To elucidate how PtdIns5P could affect actin dynamics and migration, we first focused on the Rho GTPases, which are good candidates to integrate PI signalling and cytoskeletal dynamics. To allow fine-tuning of PtdIns5P production, we developed inducible Tet-Off MEF cell lines stably expressing Myc-EGFP-IpgD (called MEF-IpgD), a bacterial phosphatase that transforms PtdIns(4,5)P 2 into PtdIns5P (ref. 13 ). As controls, inducible MEF cell lines expressing the Myc-EGFP-Inp54p phosphatase (PtdIns(4,5)P 2 5-phosphatase that produces PtdIns4P) and Myc-EGFP-IpgD C438S (a phosphatase-dead mutant called MEF-IpgD-CS) were also generated. MEF-IpgD were characterized by the production of high levels of PtdIns5P and a concomitant drop in PtdIns(4,5)P 2 ( Fig. 1a and Supplementary Fig. 1a ), reproducing what is observed with S. flexneri -infected or IpgD-expressing HeLa cells [10] , [13] , [14] . Mass assay [24] , together with confocal imaging using the GST-FYVE (Hrs) probe that binds to PtdIns3P, demonstrated that IpgD expression did not affect significantly PtdIns3P levels nor distribution ( Supplementary Fig. 1b,c ). Activation of known PtdIns5P response pathways, Akt, GSK3 and FHKR, validated the cell lines for further studies ( Supplementary Fig. 1d ) [10] , [14] . As expected, no change in PtdIns5P and PtdIns(4,5)P 2 levels nor Akt activation were observed with the MEF-IpgD-CS cell line ( Fig. 1a and Supplementary Fig. 1a,e ). 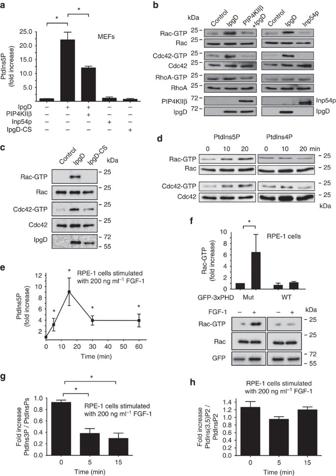Figure 1: PtdIns5P activates Rac1 and Cdc42. (a) MEF Tet-Off IpgD, Inp54p, or IpgD-CS-expressing cells were transfected or not with EGFP-PIP4KIIß. After serum starvation, PtdIns5P levels were quantified by mass assay. Data are shown as mean±s.e.m. (n=3–6; *P<0.05 using non-parametrict-test) (b) Lysates from serum-starved MEFs were subjected to pull-down experiments to monitor the levels of active Rac1, Cdc42 and RhoA. IpgD and Inp54p were detected using an anti-myc antibody and PIP4KIIß using an anti-GFP antibody. (c) Lysates from serum-starved MEFs were subjected to pull-down experiments to monitor levels of active Rac1 and Cdc42 as in (b). (d) Lysates from serum-starved MEFs, treated with the indicated exogenous-PtdInsP (15 μM) for the indicated times, were subjected to pull-down experiments as in (b). Data are representative of three to five experiments. (e) RPE-1 cells were serum-starved overnight and stimulated with 200 ng ml−1FGF-1 for the indicated time and PtdIns5P levels were quantified by mass assay. Data are shown as mean±s.e.m. (n=4; *P<0.05 using non-parametrict-test). (f) Rac1 activation was monitored by pull-down from serum-starved RPE-1 cells transduced by GFP-3xPHD wild type (WT) or GFP-3xPHD PI binding mutant (Mut)-expressing lentiviruses and treated or not with 200 ng ml−1FGF-1 for 15 min. Data are shown as mean±s.e.m. (n=3; *P<0.05 using one samplet-test for the deviation from mean value of 1 in the control group). (g) PtdIns3P levels (percentage of total PtdInsPs) in RPE-1 cells stimulated with 200 ng ml−1FGF-1. Data are shown as mean±s.e.m. (n=3; *P<0.05 using non-parametrict-test). (h) PtdIns(3,5)P2levels (percentage of total PtdInsP2s) in RPE-1 cells stimulated with 200 ng ml−1FGF-1. Data are shown as mean±s.e.m. (n=3; *P<0.05 using non-parametrict-test). Figure 1: PtdIns5P activates Rac1 and Cdc42. ( a ) MEF Tet-Off IpgD, Inp54p, or IpgD-CS-expressing cells were transfected or not with EGFP-PIP4KIIß. After serum starvation, PtdIns5P levels were quantified by mass assay. Data are shown as mean±s.e.m. ( n =3–6; * P< 0.05 using non-parametric t -test) ( b ) Lysates from serum-starved MEFs were subjected to pull-down experiments to monitor the levels of active Rac1, Cdc42 and RhoA. IpgD and Inp54p were detected using an anti-myc antibody and PIP4KIIß using an anti-GFP antibody. ( c ) Lysates from serum-starved MEFs were subjected to pull-down experiments to monitor levels of active Rac1 and Cdc42 as in ( b ). ( d ) Lysates from serum-starved MEFs, treated with the indicated exogenous-PtdInsP (15 μM) for the indicated times, were subjected to pull-down experiments as in ( b ). Data are representative of three to five experiments. ( e ) RPE-1 cells were serum-starved overnight and stimulated with 200 ng ml −1 FGF-1 for the indicated time and PtdIns5P levels were quantified by mass assay. Data are shown as mean±s.e.m. ( n =4; * P< 0.05 using non-parametric t -test). ( f ) Rac1 activation was monitored by pull-down from serum-starved RPE-1 cells transduced by GFP-3xPHD wild type (WT) or GFP-3xPHD PI binding mutant (Mut)-expressing lentiviruses and treated or not with 200 ng ml −1 FGF-1 for 15 min. Data are shown as mean±s.e.m. ( n =3; * P< 0.05 using one sample t -test for the deviation from mean value of 1 in the control group). ( g ) PtdIns3P levels (percentage of total PtdInsPs) in RPE-1 cells stimulated with 200 ng ml −1 FGF-1. Data are shown as mean±s.e.m. ( n =3; * P< 0.05 using non-parametric t -test). ( h ) PtdIns(3,5)P 2 levels (percentage of total PtdInsP 2 s) in RPE-1 cells stimulated with 200 ng ml −1 FGF-1. Data are shown as mean±s.e.m. ( n =3; * P< 0.05 using non-parametric t -test). Full size image Expression of IpgD resulted in a strong activation of both Rac1 and Cdc42, while RhoA remained stable ( Fig. 1b ). As a control, co-expression of IpgD and PIP4KIIß, which drastically reduced the amount of PtdIn5P ( Fig. 1a ), brought Rac1- and Cdc42-GTP back to control levels ( Fig. 1b ). Inp54p and IpgD-CS expressions resulted in no change in Rac1 or Cdc42 activation ( Fig. 1b,c ). Importantly, study of the F-actin confirmed that IpgD expression induced disappearance of actin stress fibres, while cortical actin was not affected. Treatment with the Rac inhibitor NSC23766 (ref. 25 ) restored F-actin polymerization, demonstrating that Rac was responsible for PtdIns5P-dependent actin remodelling ( Supplementary Fig. 2a ). Interestingly, activation of Cdc42 by PtdIns5P was not involved in F-actin dynamics inside the cell but was instrumental to cortical actin assembly since no pericellular actin staining could be seen upon treatment with secramine A [26] , a potent inhibitor of Cdc42 ( Supplementary Fig. 2a ). This observation suggested that Rac1 and Cdc42 might regulate different actin pools downstream of PtdIns5P. Time-course experiments performed on MEFs treated with short-chain PtdInsPs demonstrated that PtdIns5P was responsible for GTPase activation and F-actin breakdown ( Fig. 1d and Supplementary Fig. 2b,c ). We had previously identified class I PI 3-kinases sensitive to LY294002 inhibition as targets activated by PtdIns5P [14] . GTPases pull-downs performed in MEF-IpgD or control MEFs challenged with synthetic PtdIns5P in the presence of LY294002 demonstrated that PI 3-kinases were not responsible for Rac1 activation in this context ( Supplementary Fig. 3a,b ). Since Rac1 had the strongest impact on actin dynamics, we focused on the study of this GTPase downstream of PtdIns5P in physiological and pathological models: RPE-1 cells stimulated by FGF-1 and anaplastic lymphomas expressing the NPM-ALK oncogene. It was recently shown that FGF-1 stimulated 2D migration of BJ foreskin fibroblasts by producing PtdIns5P through a signalling cascade that involved the class III PI 3-kinase Vps34, PIKfyve and the MTMR3 myotubularin [15] , [27] . We therefore checked whether PtdIns5P was a feature of FGF-1 stimulation by measuring PtdIns5P production in RPE-1 cells. When challenged with FGF-1, an important transitory increase in PtdIns5P peaking at 15 min of stimulation was observed ( Fig. 1e ). FGF-1 also induced activation of Rac1 in a PtdIns5P-dependent way since sequestration of this PI with the trapping probe GFP-3xPHD [8] , [10] dropped Rac1-GTP back to control levels ( Fig. 1f ). To go further into deciphering the metabolic pathway of PdIns5P upon FGF-1 stimulation, RPE-1 cells were metabolically labelled with [ 32 P]orthophosphate before stimulation. A significant drop in PtdIns3P amounts was observed after 5–15 min of treatment, while levels of PtdIns(3,5)P 2 and other PIs were hardly affected ( Fig. 1g,h ). This suggested that PtdIns3P could be a precursor of PtdIns5P synthesis through transformation into PtdIns(3,5)P 2 by PIKfyve and subsequent dephosphorylation by a 3-Phosphatase as demonstrated by Oppelt et al. [15] in BJ fibroblasts. The lack of a concomitant decrease in PtdIns(3,5)P 2 could reflect a rapid and transient metabolization difficult to assess with such an elusive PI. However, these observations do not rule out the possibility that PtdIns5P could come from the action of PIKfyve on PtdIns. The impact of PtdIns5P on Rho GTPases was also analysed in a pathological context by studying anaplastic large-cell lymphomas expressing the NPM-ALK tyrosine kinase oncogene. We previously demonstrated that NPM-ALK(+) cells had elevated levels of PtdIns5P, which could be attributed to activation of PIKfyve by the oncogene in NPM-ALK-expressing NIH-3T3 fibroblasts [21] , [28] . We used the Cost and Karpas 299 patient-derived cell lines and showed by treatment with the YM201636 inhibitor and shRNA depletion that PIKfyve was responsible for the increase in PtdIns5P in these cells ( Fig. 2a,b ). Treatment with the YM201636 inhibitor, PIKfyve shRNA, or expression of GFP-3xPHD, clearly demonstrated that PtdIns5P production was also responsible for Rac1 activation in NPM-ALK(+) cells ( Fig. 2c–e ). Together, these data demonstrate that PtdIns5P-induced activation of Rho GTPases and the subsequent modulation of actin dynamics are prevalent mechanisms observed in different models. 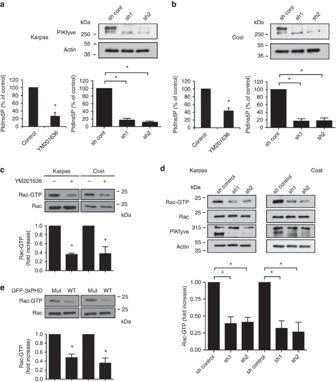Figure 2: PtdIns5P is essential for Rac activation in NPM-ALK(+) cells. (a) PtdIns5P mass levels in serum-starved Karpas 299 treated overnight or not with 800 nM of the PIKfyve inhibitor YM201636 or transduced with lentiviruses expressing shRNA directed against PIKfyve (sh1 and sh2). Data are shown as mean±s.e.m. (n=3 (Karpas 299 cells);n=3 (Cost cells); *P<0.05 using one samplet-test for the deviation from mean value of 100 in the control group). (b) Same experiment as in (a) with Cost cells. (c) Rac1 activation was monitored by pull-down from serum-starved Karpas 299 and Cost cells treated overnight or not with 800 nM YM201636. (d) Rac1 activation was monitored by pull-down from serum-starved Karpas 299 and Cost cells stably expressing shRNA directed against PIKfyve (sh1 and sh2). Data are shown as mean±s.e.m. (n=3; *P<0.05 using one samplet-test for the deviation from mean value of 1 in the control group). (e) Rac1 activation was monitored by pull-down from serum-starved Karpas 299 and Cost cells transduced by GFP-3xPHD wild type (WT) or GFP-3xPHD PI binding mutant (Mut)-expressing lentiviruses. Data are shown as mean±s.e.m. (n=3; *P<0.05 using one samplet-test for the deviation from mean value of 1 in the control group). Figure 2: PtdIns5P is essential for Rac activation in NPM-ALK(+) cells. ( a ) PtdIns5P mass levels in serum-starved Karpas 299 treated overnight or not with 800 nM of the PIKfyve inhibitor YM201636 or transduced with lentiviruses expressing shRNA directed against PIKfyve (sh1 and sh2). Data are shown as mean±s.e.m. ( n =3 (Karpas 299 cells); n =3 (Cost cells); * P< 0.05 using one sample t -test for the deviation from mean value of 100 in the control group). ( b ) Same experiment as in ( a ) with Cost cells. ( c ) Rac1 activation was monitored by pull-down from serum-starved Karpas 299 and Cost cells treated overnight or not with 800 nM YM201636. ( d ) Rac1 activation was monitored by pull-down from serum-starved Karpas 299 and Cost cells stably expressing shRNA directed against PIKfyve (sh1 and sh2). Data are shown as mean±s.e.m. ( n =3; * P< 0.05 using one sample t -test for the deviation from mean value of 1 in the control group). ( e ) Rac1 activation was monitored by pull-down from serum-starved Karpas 299 and Cost cells transduced by GFP-3xPHD wild type (WT) or GFP-3xPHD PI binding mutant (Mut)-expressing lentiviruses. Data are shown as mean±s.e.m. ( n =3; * P< 0.05 using one sample t -test for the deviation from mean value of 1 in the control group). Full size image The RacGEF Tiam1 is activated upon PtdIns5P elevation Rho GTPases cycle between an inactive GDP-bound and an active GTP-bound state with the assistance of GEFs, which are required for proper local GTPase activation [29] . The Rac inhibitor NSC23766 blocks interaction between Rac1 and a subset of its GEFs, namely Tiam1 and Trio [25] . Tiam1 is specific for Rac1 in vivo and has been involved in Rac1-induced cytoskeleton remodelling, motility and invasion in many different cell types [30] , [31] . Interestingly, pull-down experiments with the nucleotide free mutant GST-Rac1 G15A , which display high affinity for active GEFs, demonstrated that Tiam1 was activated upon PtdIns5P elevation in FGF-1-treated RPE-1 cells and MEF-IpgD, whereas an unrelated GEF for RhoA (p115 RhoGEF) was not. Accordingly, pre-treatment of cells with NSC23766 abolished Tiam1 association to Rac G15A ( Fig. 3a,b ). Subcellular fractionation of control MEFs, MEF-IpgD or MEF-Inp54p confirmed that the relocation of Tiam1 to the heavy membrane fraction that marked its activation was only observed upon IpgD expression ( Supplementary Fig. 4a ). The GST-Cdc42 G15A mutant did not pull down any active Tiam1 (not shown). Rac1 G15A pull-downs also demonstrated that Tiam1 was activated in NPM-ALK(+) anaplastic lymphomas ( Fig. 3c ). The NPM-ALK inhibitor WHI-154 prevented Tiam1 from binding to Rac1 G15A in both Karpas 299 and Cost cells, indicating that the oncogene was responsible for Tiam1 activation ( Fig. 3c ). Tiam1 was previously identified as part of the proteomic signature of NPM-ALK, reinforcing the idea of its involvement in NPM-ALK-mediated tumorigenicity [32] . Immunoprecipitations confirmed that Tiam1 was a binding partner of the oncogene ( Supplementary Fig. 4b ), and demonstrated that it was a tyrosine phosphorylation target of NPM-ALK ( Supplementary Fig. 4c ). 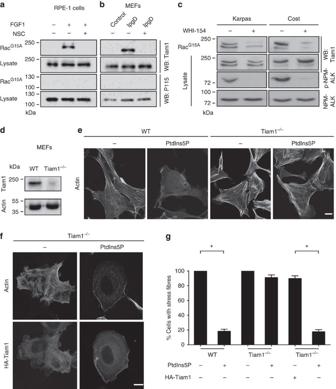Figure 3: PtdIns5P elevation activates Tiam1, which is required for actin dynamics. (a) GEF trapping assays using GST-Rac1G15Aagarose beads were performed on serum-starved RPE-1 cells stimulated or not with 200 ng ml−1FGF-1 for 15 min and treated or not with NSC23766. Tiam1 and p115 RhoGEF binding were detected by western blotting. (b) Same experiment as in (a) performed on serum-starved MEF cells. (c) Same experiments as in (a) carried out on serum-starved Karpas 299 and Cost cells treated overnight or not with 15 μM WHI-154. Lysates were probed with anti-Tiam1, anti-P-NPM-ALK(Y664) or anti-ALK (Sp8) antibodies. (d) Lysates from primary WT and Tiam1−/−MEF cells were subjected to western blot analysis with anti-Tiam1. (e) Serum-starved primary WT and Tiam1−/−MEFs were treated or not with exogenous PtdIns5P (15 μM) for 30 min. Cells were then fixed and the actin cytoskeleton was visualized by staining with AlexaFluor 488-phalloidin. Scale bar, 10 μm. (f) Serum-starved primary WT and Tiam1−/−MEFs transfected with HA-Tiam1 were treated with exogenous PtdIns5P (15 μM) for 30 min. Cells were then fixed and the actin cytoskeleton was visualized by staining with AlexaFluor 488-phalloidin and Tiam1 with and HA antibody. Scale bar, 10 μm. (g) Quantitative analysis of the experiment described in (e) and (f). Data are shown as mean±s.e.m. (n=3; *P<0.05 using one samplet-test for the deviation from mean value of 100 in the control group and using non-parametric one way ANOVA (Kruskal–Wallis) with Dunn’s post test). Figure 3: PtdIns5P elevation activates Tiam1, which is required for actin dynamics. ( a ) GEF trapping assays using GST-Rac1 G15A agarose beads were performed on serum-starved RPE-1 cells stimulated or not with 200 ng ml −1 FGF-1 for 15 min and treated or not with NSC23766. Tiam1 and p115 RhoGEF binding were detected by western blotting. ( b ) Same experiment as in ( a ) performed on serum-starved MEF cells. ( c ) Same experiments as in ( a ) carried out on serum-starved Karpas 299 and Cost cells treated overnight or not with 15 μM WHI-154. Lysates were probed with anti-Tiam1, anti-P-NPM-ALK(Y664) or anti-ALK (Sp8) antibodies. ( d ) Lysates from primary WT and Tiam1 −/− MEF cells were subjected to western blot analysis with anti-Tiam1. ( e ) Serum-starved primary WT and Tiam1 −/− MEFs were treated or not with exogenous PtdIns5P (15 μM) for 30 min. Cells were then fixed and the actin cytoskeleton was visualized by staining with AlexaFluor 488-phalloidin. Scale bar, 10 μm. ( f ) Serum-starved primary WT and Tiam1 −/− MEFs transfected with HA-Tiam1 were treated with exogenous PtdIns5P (15 μM) for 30 min. Cells were then fixed and the actin cytoskeleton was visualized by staining with AlexaFluor 488-phalloidin and Tiam1 with and HA antibody. Scale bar, 10 μm. ( g ) Quantitative analysis of the experiment described in ( e ) and ( f ). Data are shown as mean±s.e.m. ( n =3; * P< 0.05 using one sample t -test for the deviation from mean value of 100 in the control group and using non-parametric one way ANOVA (Kruskal–Wallis) with Dunn’s post test). Full size image Moreover, ectopic expression of IpgD in Tiam1 −/− primary MEFs ( Fig. 3d ) in which the GEF had been knocked out [33] as well as exogenous PtdIns5P stimulation of WT MEFs pre-treated with NSC23766 failed to activate Rac1, showing that Tiam1 is essential for Rac1 activation in response to PtdIns5P elevation ( Supplementary Fig. 4d,e ). Importantly, PtdIns5P-elicited F-actin breakdown was totally abolished in Tiam1 −/− MEFs, which conserved strong actin fibres ( Fig. 3e,g ). Re-expression of Tiam1 in Tiam1 −/− MEFs restored PtdIns5P-dependent F-actin disappearance, confirming that Tiam1 was responsible for this effect ( Fig. 3f,g ). The known NPM-ALK-dependent actin disassembly that was previously shown to be regulated by Rac [18] , was also blocked when NPM-ALK was expressed in Tiam1 −/− MEFs, as shown by the persistence of actin fibres ( Supplementary Fig. 4f ). Of note, NPM-ALK-expressing Tiam1 −/− MEF exhibited filopodia, suggesting that activation of Cdc42 downstream of the oncogene was maintained in the absence of Tiam1 ( Supplementary Fig. 4f , white arrows). In agreement with the lack of NPM-ALK-dependent actin fibres remodelling in Tiam1 −/− cells, the invasion elicited by expression of the oncogene was blocked in Tiam1 −/− MEF ( Supplementary Fig. 4g ). Together, these data point to PtdIns5P acting on the Tiam1/Rac1 module as a general way of eliciting actin remodelling in various cell systems. Tiam1 PHc preferentially binds to PtdIns5P Tiam1 has the particularity of bearing two PH domains. While the N-terminal domain (PHn) seems to be critical for protein interactions and Tiam1 localization, the PHc domain, contained in the catalytic DH-PH region, is responsible for Tiam1 exchange activity [34] , [35] ( Fig. 4a ). It had been previously reported that the PHc domain displayed affinity for PtdIns3P (ref. 36 ). We used recombinant GST-DH-PHc to probe PIP strips and PIP arrays (serial dilution of various PIPs) to check whether it had affinity for other PIs. These experiments not only confirmed that Tiam1 PHc bound to PtdIns3P but also revealed that it displayed a stronger affinity for PtdIns5P ( Fig. 4b,c ), whereas Tiam1 PHn preferentially bound to PtdIns(4,5)P 2 and PtdIns(3,4,5)P 3 ( Fig. 4d and ref. 37 ). Lysines from both variable loops L1 (ß1/ß2) and L2 (ß2/ß3) of the Tiam1 PHc have been shown to be required for PtdIns3P binding [36] ( Fig. 4a ). We repeated the experiments using mutants where the lysines were substituted by glutamines and demonstrated that those residues were important for binding to both PtdIns3P and PtdIns5P ( Fig. 4c ). Sedimentation assays with liposomes containing a mix of PC:PE and either PtdIns3P, PtdIns4P or PtdIns5P confirmed that GST-DH-PHc-Tiam1 only bound liposomes bearing either PC:PE:PtdIns3P or PC:PE:PtdIns5P ( Fig. 4e ). The stronger binding to PtdIns5P-containing liposomes confirmed that Tiam1 PHc preferentially interacted with PtdIns5P. 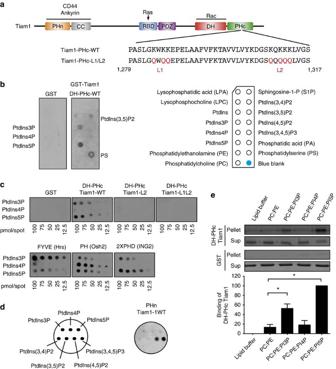Figure 4: The C-terminal PH domain of Tiam1 binds to PtdIns5P. (a) Structure of the Tiam1 protein. PHn, N-terminal pleckstrin homology domain; CC, coiled-coil region; RBD, Ras-binding domain; PDZ, postsynaptic density-96/Discs large/Zonaoccludens-1; DH, Dbl homology domain (the catalytic domain); PHc, C-terminal pleckstrin homology domain. Amino-acid sequence of Tiam1 PHc-WT and mutants are presented below. Lysine to glutamine mutations in PH*L2 and PH*L1/L2 are in red. (b) GST or GST-Tiam1-DH-PHc (0.5 μg ml−1) was used to probe PIP array. Weak binding to phosphatidylserine was sometimes observed but was not reproduced in all experiments. Data are representative of more than five experiments done with commercial or homemade membranes. (c) A total of 0.5 μg ml−1of each GST-tagged protein was used to probe nitrocellulose spotted with serial dilutions of PtdIns3P, PtdIns4P and PtdIns5P, as described under ‘Methods’. Lipid–protein overlays are representative of five independent experiments. (d) A total of 0.5 μg ml−1of GST-tagged PHn of Tiam1 was used to probe nitrocellulose spotted with 100 pmol of each PI as described under ‘Methods’. The result is representative of three independent experiments. (e) GST or Tiam1 GST-DH-PHc was incubated with liposomes containing the indicated PIs. Liposomes were recovered by centrifugation and protein content was analysed by SDS-PAGE and silver staining. Bottom panel: quantitative analysis of liposome binding experiments. Results are presented as mean±s.e.m. (n=3; *P<0.05 using one samplet-test for the deviation from mean value of 100 in the PI5P group and using non-parametrict-test). Figure 4: The C-terminal PH domain of Tiam1 binds to PtdIns5P. ( a ) Structure of the Tiam1 protein. PH n , N-terminal pleckstrin homology domain; CC, coiled-coil region; RBD, Ras-binding domain; PDZ, postsynaptic density-96/Discs large/Zonaoccludens-1; DH, Dbl homology domain (the catalytic domain); PHc, C-terminal pleckstrin homology domain. Amino-acid sequence of Tiam1 PHc-WT and mutants are presented below. Lysine to glutamine mutations in PH*L2 and PH*L1/L2 are in red. ( b ) GST or GST-Tiam1-DH-PHc (0.5 μg ml −1 ) was used to probe PIP array. Weak binding to phosphatidylserine was sometimes observed but was not reproduced in all experiments. Data are representative of more than five experiments done with commercial or homemade membranes. ( c ) A total of 0.5 μg ml −1 of each GST-tagged protein was used to probe nitrocellulose spotted with serial dilutions of PtdIns3P, PtdIns4P and PtdIns5P, as described under ‘Methods’. Lipid–protein overlays are representative of five independent experiments. ( d ) A total of 0.5 μg ml −1 of GST-tagged PHn of Tiam1 was used to probe nitrocellulose spotted with 100 pmol of each PI as described under ‘Methods’. The result is representative of three independent experiments. ( e ) GST or Tiam1 GST-DH-PHc was incubated with liposomes containing the indicated PIs. Liposomes were recovered by centrifugation and protein content was analysed by SDS-PAGE and silver staining. Bottom panel: quantitative analysis of liposome binding experiments. Results are presented as mean±s.e.m. ( n =3; * P< 0.05 using one sample t -test for the deviation from mean value of 100 in the PI5P group and using non-parametric t -test). Full size image PtdIns5P stimulates Tiam1 DH-PHc activity in vitro We next analysed the effect of PtdIns5P on the intrinsic Tiam1 GEF activity by performing in vitro nucleotide exchange assays using recombinant Rac1 loaded with bodipy-FL-GDP. It has been previously reported that the DH-PHc of Tiam1 displayed a much better activity on prenylated Rac-GDP bound to liposomes versus non prenylated soluble Rac-GDP [36] , [38] . These observations suggested that anchoring of Rac-GDP to membranes was important for proper presentation of the GTPase to the DH-PH domain. Rearrangement of the DH-PH structure following association with PtdInsP would then stimulate GDP to GTP exchange. We then used the findings of a recent study by Malecka et al. [39] to adapt a system that mimics the prenylation-dependent membrane anchoring of GTPases by creating liposomes containing PC, PE and lipids bearing a modified Ni 2+ -NTA head group (DGS-NTA(Ni)) capable of binding to a recombinant C-terminal hexahistidine-tagged version of Rac1 ( Fig. 5a ). Sedimentation assays confirmed approximately stoichiometric binding of Rac1-His to the Ni 2+ -NTA lipid exposed on the liposomes’ outer surface [39] ( Fig. 5b ). We then performed exchange assays using liposomes bearing different PtdInsP species and Rac1-His loaded with bodipy FL-GDP in the presence of soluble Tiam1 DH-PHc. Maximum exchange activity was achieved by adding EDTA to the reaction, while spontaneous Rac1 exchange was assessed in the presence of buffer only. In the presence of PtdIns5P-bearing liposomes, we observed a strong Tiam1 exchange activity, while PtdIns4P had no effect ( Fig. 5c,d ). In this assay, we also observed a weak increase in Tiam1 exchange activity in the presence of PtdIns3P-bearing liposomes, demonstrating that both PtdIns3P and PtdIns5P could potentiate Tiam1 activity in vitro ( Fig. 5c,d ). Our observations demonstrate the potency of this assay that mimics membrane and proteins functional interactions. These results suggest that Tiam1 recruitment by PtdIns5P is sufficient to increase intrinsic Tiam1 exchange activity. 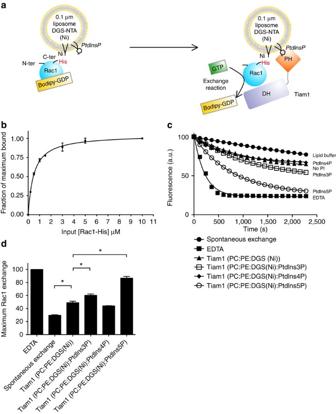Figure 5: PtdIns5P increases Tiam1 DH-PHc intrinsic exchange activity. (a) The assay was performed on 0.1 μm of Ni2+-NTA-containing liposomes (with the different PI species) bound to Rac-His loaded with Bodipy FL-GDP. Recombinant Tiam1 DH-PHc was added and the nucleotide exchange reaction was started by adding an excess of GTP. The exchange reaction was followed by fluorospectroscopy. (b) Rac1-His-binding capacity of Ni2+-NTA-containing liposomes. A total of 300 μM liposomes PC:PE:PEfluorescein:DGS-NTA(Ni) (67:28:2:3 molar ratio) were incubated with increasing concentrations of Rac1-His. Liposome-associated Rac1-His was quantified by SDS–PAGE followed by Coomassie staining and plotted as a function of Rac-His input concentration using ImageJ. Data are shown as mean±s.e.m. (n=3 experiments). (c) Recombinant Rac1-His loaded with Bodipy FL-GDP (1 μM final) was bound to liposomes via DGS-NTA(Ni). Liposomes were composed of PC:PE:DGS-NTA(Ni):PI (61:30:3:6 molar ratio). DH-PHc Tiam1 (100 nM) was then preincubated and the exchange reaction (Bodipy FL-GDP/GTP) was started by adding 200 μM final GTP. The data were fit as a single exponential decay and all experiments were performed three times with identical results. (d) Quantification of the experiment described in (c). Results are expressed as maximum Rac1 exchange att=40 min assuming 100% exchange was obtained with EDTA. Data are shown as mean±s.e.m. (n=3; *P<0.05 using non-parametrict-test) Figure 5: PtdIns5P increases Tiam1 DH-PHc intrinsic exchange activity. ( a ) The assay was performed on 0.1 μm of Ni 2+ -NTA-containing liposomes (with the different PI species) bound to Rac-His loaded with Bodipy FL-GDP. Recombinant Tiam1 DH-PHc was added and the nucleotide exchange reaction was started by adding an excess of GTP. The exchange reaction was followed by fluorospectroscopy. ( b ) Rac1-His-binding capacity of Ni 2+ -NTA-containing liposomes. A total of 300 μM liposomes PC:PE:PE fluorescein :DGS-NTA(Ni) (67:28:2:3 molar ratio) were incubated with increasing concentrations of Rac1-His. Liposome-associated Rac1-His was quantified by SDS–PAGE followed by Coomassie staining and plotted as a function of Rac-His input concentration using ImageJ. Data are shown as mean±s.e.m. ( n =3 experiments). ( c ) Recombinant Rac1-His loaded with Bodipy FL-GDP (1 μM final) was bound to liposomes via DGS-NTA(Ni). Liposomes were composed of PC:PE:DGS-NTA(Ni):PI (61:30:3:6 molar ratio). DH-PHc Tiam1 (100 nM) was then preincubated and the exchange reaction (Bodipy FL-GDP/GTP) was started by adding 200 μM final GTP. The data were fit as a single exponential decay and all experiments were performed three times with identical results. ( d ) Quantification of the experiment described in ( c ). Results are expressed as maximum Rac1 exchange at t =40 min assuming 100% exchange was obtained with EDTA. Data are shown as mean±s.e.m. ( n =3; * P< 0.05 using non-parametric t -test) Full size image PtdIns5P, Tiam1 and Rac1 localize on endosomes within ruffles We then investigated the localization of PtdIns5P, Tiam1 and Rac1, knowing that PtdIns5P produced by IpgD expression in HeLa and BHK cells rapidly accumulates on early endosomes [10] . We focused on MEF-IpgD as a model because they are easy to image and IpgD-elicited increase in PtdIns5P recapitulated Tiam1/Rac1 activation and actin dynamics observed in other models (this and other studies [10] , [13] , [14] , [21] , [28] ). Cells were seeded on fibronectin micropatterns, which mimics the restrained adhesion geometry cells encounter within tissues, permitting enhanced monitoring of better membrane dynamics [40] . Cells plated onto crossbow micropatterns adopted a polarized shape with a lamellipodium at the front ( Supplementary Fig. 5 ). MEF-IpgD exhibited a strong dorsal and peripheral ruffling activity and extended large lamellipodia to probe the matrix surrounding the micropattern ( Supplementary Fig. 5a , left panel). Time-lapse experiments demonstrated that ruffling was polarized ( Supplementary Fig. 5a and Supplementary Movies 1 and 2 ). Plating on circular micropatterns led to a loss of polarization, but MEF-IpgD retained a strong ruffling activity around the cell body ( Supplementary Fig. 5a , right panel, and Supplementary Movies 3 and 4 ). PtdIns5P was visualized using the GST-2xPHD probe. PtdIns5P decorates intracellular vesicles localized at the foot of dorsal ruffles, sites with strong actin dynamics as shown by phalloidin staining, reinforcing the idea of a functional link between PtdIns5P, trafficking and ruffle formation ( Supplementary Fig. 5b , zooms). Confocal microscopy demonstrated that Tiam1, Rac1 and PtdIns5P partially colocalized with vesicles positive for EEA1, a marker of early endosomes, suggesting that PtdIns5P was recruiting the Tiam1/Rac1 module on these vesicles ( Fig. 6a,b ). As protein–protein association can be very transient and colocalization of several partners impaired by sterical hindrance on small structures such as vesicles, we also performed a Proximity Ligation Assay (Duolink) demonstrated to be more sensitive to study those type of interactions [41] . This analysis confirmed the data obtained by immunofluorescence staining ( Supplementary Fig. 6 ). Weak colocalization could also be detected in control MEFs at structures where basal levels of PtdIns5P were present ( Supplementary Fig. 7a , line scans a and d). Study of Cdc42 localization demonstrated that it was mostly located at the plasma membrane in MEF-IpgD ( Supplementary Fig. 7b ). 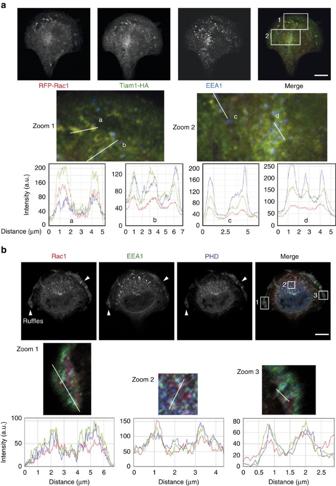Figure 6: PtdIns5P localizes to early endosomes with Tiam1 and Rac1. (a) MEF-IpgD were co-transfected with mRFP-Rac1 and Tiam1-HA before induction of IpgD expression. Cells were then serum-starved, fixed and stained for EEA1 and the HA tag. The lower panels (zoom 1 and zoom 2) represent high magnifications of areas 1 and 2 shown on the upper merge panel. On each zoom, the two lines drawn across the cells indicate the path of a 3-pixel-wide linescan (zoom 1: a,b, zoom 2: c,d). Respective line scans are shown below zoom panels. (b) Serum-starved MEF-IpgD were stained for endogenous Rac1, EEA1 and PtdIns5P (using the GST-2xPHD probe). Arrowheads indicate zones of ruffling. Magnifications of areas 1, 2 and 3 shown as boxes in the merged image, as well as their respective linescans (3-pixels wide) are shown at the bottom of the panel. Scale bar, 10 μm. Figure 6: PtdIns5P localizes to early endosomes with Tiam1 and Rac1. ( a ) MEF-IpgD were co-transfected with mRFP-Rac1 and Tiam1-HA before induction of IpgD expression. Cells were then serum-starved, fixed and stained for EEA1 and the HA tag. The lower panels (zoom 1 and zoom 2) represent high magnifications of areas 1 and 2 shown on the upper merge panel. On each zoom, the two lines drawn across the cells indicate the path of a 3-pixel-wide linescan (zoom 1: a,b, zoom 2: c,d). Respective line scans are shown below zoom panels. ( b ) Serum-starved MEF-IpgD were stained for endogenous Rac1, EEA1 and PtdIns5P (using the GST-2xPHD probe). Arrowheads indicate zones of ruffling. Magnifications of areas 1, 2 and 3 shown as boxes in the merged image, as well as their respective linescans (3-pixels wide) are shown at the bottom of the panel. Scale bar, 10 μm. Full size image While re-expression of WT Tiam1 restored F-actin breakdown in Tiam1 −/− MEFs, expression of the Tiam1-L1L2 mutant that cannot bind PtdIns5P was not capable of remodelling actin upon PtdIns5P increase ( Fig. 7 ). Morphological analysis demonstrated that overexpression of WT Tiam1 together with PtdIns5P treatment resulted in the appearance of enlarged vesicles positive for EEA1, suggesting that they worked together to affect trafficking. Accordingly, overexpression of Tiam1 L1L2 did not affect the structure of EEA1 endosomes, demonstrating that Tiam1 binding to PtdIns5P was mandatory for this effect to occur ( Fig. 7 , zooms). In line with this observation, Tiam1 L1L2 was not recruited to EEA1 endosomes as was WT-Tiam1 ( Fig. 7 , zooms and linescans). 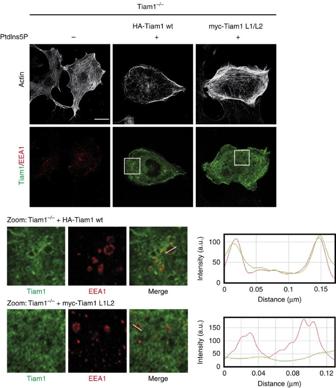Figure 7: Tiam1 binding to PtdIns5P drives F-actin remodelling and localization to EEA1 endosomes. Serum-starved primary Tiam1−/−MEF transfected with HA-Tiam1 or myc-Tiam1 L1L2 were treated with exogenous PtdIns5P (15 μM) for 30 min. Cells were then fixed and the actin cytoskeleton was visualized by staining with AlexaFluor 488-phalloidin and Tiam1 with HA or myc antibodies. Scale bar, 10 μm. The lower panels represent higher magnifications for indicated areas shown as boxes in the merged image, as well as their respective linescans (3-pixels wide). Figure 7: Tiam1 binding to PtdIns5P drives F-actin remodelling and localization to EEA1 endosomes. Serum-starved primary Tiam1 −/− MEF transfected with HA-Tiam1 or myc-Tiam1 L1L2 were treated with exogenous PtdIns5P (15 μM) for 30 min. Cells were then fixed and the actin cytoskeleton was visualized by staining with AlexaFluor 488-phalloidin and Tiam1 with HA or myc antibodies. Scale bar, 10 μm. The lower panels represent higher magnifications for indicated areas shown as boxes in the merged image, as well as their respective linescans (3-pixels wide). Full size image Taken together, these data favour the hypothesis that PtdIns5P enrichment in early endosomes recruits and locally activates the Tiam1/Rac1 module to drive targeted actin and membrane dynamics. PtdIns5P regulates Rac1 activity in ruffles and vesicles Active Rac1 has been reported to localize in ruffles and early endosomes, where we demonstrated PtdIns5P to be enriched in several cell types [10] , [13] , [42] . Indeed, Rac1 is a pivotal regulator of actin dynamics, which drives the formation of membrane protrusions such as lamellipodia, peripheral and dorsal circular ruffles (unique sites where spatially restricted actin remodelling controls cellular motility). Observation of Rac1 localization over time by monitoring the CFP fluorescence of Raichu-Rac1 demonstrated that Rac1 was not only present on early endosomes ( Fig. 8a ) but also relocated to ruffles when levels of PtdIns5P increased ( Fig. 8a ). Dynamic analysis revealed that CFP-Rac1-containing dorsal ruffles moved towards the edge of the lamellipodium before being engulfed, illustrating the polarization of this process ( Fig. 8a , zoom and kymograph). We then recorded FRET (Förster Resonance Energy Transfer) emitted by the Raichu-Rac1 biosensor over time to monitor local activity of the Tiam1/Rac1 module [43] . When MEF-IpgD were spatially restricted on micropatterns, active Rac1 could be observed at the cell periphery and in circular ruffles that were moving along the lamellipodium ( Figs 8b and 9c , and Supplementary Movie 5 ). When plated on non-patterned fibronectin, cells spread out on the coverslips and extend lamellipodia, resulting in a lower rate of ruffling [44] , and therefore facilitating FRET imaging of discrete internal structures such as vesicles. Real-time imaging of non-patterned cells revealed that Rac1 was also active on small vesicles that were moving within the lamellipodium ( Figs 8c and 9b , and Supplementary Movie 6 ). When MEFs were not challenged with PtdIns5P, Raichu-Rac1 fluorescence was largely cytosolic and no activation could be detected over time ( Figs 8d and 9c , Supplementary Fig. 8a , and Supplementary Movies 7 and 8 ). Again, monitoring of FRET activity in Tiam1 −/− MEFs demonstrated that no activation of Raichu-Rac1 was detected in the absence of GEF when PtdIns5P was added to the cells ( Figs 8e and 9c , and Supplementary Movie 9 ). 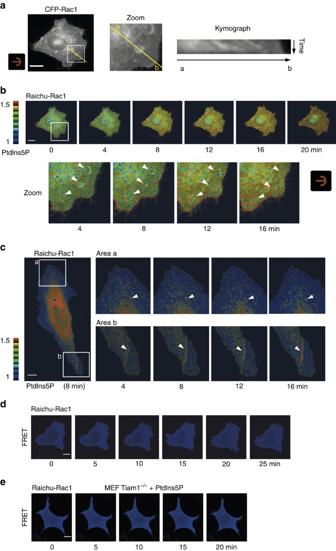Figure 8: PtdIns5P induces Rac1 activation in dorsal ruffles and vesicles. (a) MEF cells transfected with the Raichu-Rac1 encoding vector were plated on micropatterns of fibronectin and serum-starved for 6 h. Exogenous PtdIns5P was added (0.5 μM) and cells were imaged every 4 min during 20 min. Rac1 localization was visualized by monitoring CFP fluorescence. Rac1-enriched ruffles are visible on the dorsal side of the cells. On the right side, a kymograph assembled along the lamellipodium shows the dynamic towards the front of the cell. (b) Rac1 activation is visualized by color-coded FRET. High ratio values (red) correlate with higher Rac1 activity in ruffles and at the cell periphery. The lower panels represent higher magnifications for areas at the indicated time points. Arrowheads represent circular ruffles moving towards the front of the lamellipodium. (c) Similar experiments as in (b) except that no micropattern was used. The right panels represent higher magnifications of boxed areas a and b depicted on the larger image. Arrowheads indicate vesicles (area a) and ruffles (area b) with active Rac1. (d) Similar experiment as in (c) except that no PtdIns5P was added to the cells. (e) Similar experiment as in (c) except that it was performed on Tiam1−/−MEFs challenged with PtdIns5P. Scale bar, 10 μm. See alsoSupplementary Movies 5–9. Figure 8: PtdIns5P induces Rac1 activation in dorsal ruffles and vesicles. ( a ) MEF cells transfected with the Raichu-Rac1 encoding vector were plated on micropatterns of fibronectin and serum-starved for 6 h. Exogenous PtdIns5P was added (0.5 μM) and cells were imaged every 4 min during 20 min. Rac1 localization was visualized by monitoring CFP fluorescence. Rac1-enriched ruffles are visible on the dorsal side of the cells. On the right side, a kymograph assembled along the lamellipodium shows the dynamic towards the front of the cell. ( b ) Rac1 activation is visualized by color-coded FRET. High ratio values (red) correlate with higher Rac1 activity in ruffles and at the cell periphery. The lower panels represent higher magnifications for areas at the indicated time points. Arrowheads represent circular ruffles moving towards the front of the lamellipodium. ( c ) Similar experiments as in ( b ) except that no micropattern was used. The right panels represent higher magnifications of boxed areas a and b depicted on the larger image. Arrowheads indicate vesicles (area a) and ruffles (area b) with active Rac1. ( d ) Similar experiment as in ( c ) except that no PtdIns5P was added to the cells. ( e ) Similar experiment as in ( c ) except that it was performed on Tiam1 −/− MEFs challenged with PtdIns5P. Scale bar, 10 μm. See also Supplementary Movies 5–9 . 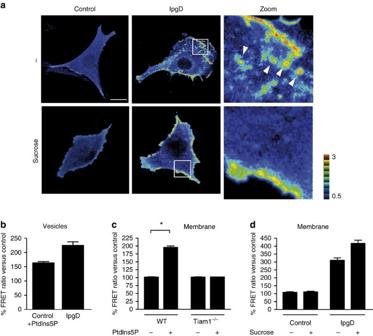Figure 9: PtdIns5P-induced localization of active Rac1 in dorsal ruffles and vesicles requires endocytosis. (a) Control and IpgD-MEF-expressing Raichu-Rac1 were serum-starved for 2 h before the addition of 0.4 M sucrose for 2 more hours. Cells were fixed and imaged. The right panels represent higher magnifications of boxed areas on the larger image. Arrowheads indicate vesicles with active Rac1. Scale bar, 10 μm. (b) Changes in FRET were represented as a percentage of FRET in vesicles over FRET in the cytosol (called ‘control’) of indicated cells and treatment. (c) Similar representation as in (b) performed on the cell periphery (plasma membrane for all; plasma membrane and ruffles in the case of WT MEFs treated by PtdIns5P). (d) Similar representation as in (b) performed on the experiment described in (a). Full size image Figure 9: PtdIns5P-induced localization of active Rac1 in dorsal ruffles and vesicles requires endocytosis. ( a ) Control and IpgD-MEF-expressing Raichu-Rac1 were serum-starved for 2 h before the addition of 0.4 M sucrose for 2 more hours. Cells were fixed and imaged. The right panels represent higher magnifications of boxed areas on the larger image. Arrowheads indicate vesicles with active Rac1. Scale bar, 10 μm. ( b ) Changes in FRET were represented as a percentage of FRET in vesicles over FRET in the cytosol (called ‘control’) of indicated cells and treatment. ( c ) Similar representation as in ( b ) performed on the cell periphery (plasma membrane for all; plasma membrane and ruffles in the case of WT MEFs treated by PtdIns5P). ( d ) Similar representation as in ( b ) performed on the experiment described in ( a ). Full size image No Rac1 activation was either observed in serum-starved control MEFs, while IpgD-MEFs displayed a strong FRET signal in ruffles and vesicles ( Fig. 9a,b and d ). To investigate the role of endocytosis in Rac1 activity in ruffles and vesicles, cells were treated with sucrose. After 2 h of treatment to allow cells to adapt to the hypertonic medium generated by the addition of sucrose, transferrin and dextran intakes were monitored. As shown in Supplementary Fig. 8b , endocytosis of both compounds was blocked. No change in FRET activity was detected upon sucrose treatment of control MEFs. However, Raichu-Rac1 activation was only detected at the periphery of IpgD-MEFs, implying that endocytosis and subsequent trafficking were required to relocate Rac1 and induce ruffling activity ( Fig. 9a,d ). FRET activity was even greater at the plasma membrane of sucrose-treated IpgD-MEFs, suggesting that IpgD-produced PtdIns5P was probably found in endosomes as a result of endocytosis ( Fig. 9d ). Altogether, those observations demonstrated that PtdIns5P recruits Tiam1 at specific sites where actin and membrane dynamics were increased due to subsequent activation of Rac1. PtdIns5P triggers and drives invasive behaviour Rac1 regulates chemotaxis in response to growth factors such as EGF, PDGF, HGF or serum via formation of lamellipodia and dorsal ruffles driven by actin dynamics [44] , [45] . As already mentioned, FGF-1 has been shown to elicit 2D migration through PIKfyve/MTMR3-dependent production of PtdIns5P (ref. 15 ). Herein, we demonstrated that the invasion through dense 3D-Matrigel by RPE-1 cells challenged by a 10% serum gradient could be recapitulated by an FGF-1 gradient ( Fig. 10a ). Interestingly, while PtdIns5P trapping with GFP-3xPHD did not affect invasion towards serum, FGF-1-dependent invasion was abrogated ( Fig. 10a ). Accordingly, NSC23766 treatment had the same effect on RPE-1 cells ( Fig. 10b ). Similar observations were made in Cost and Karpas 299 cells, where invasiveness was tested towards a gradient of FBS and SDF1α, demonstrating that the PtdIns5P/Tiam1/Rac1 module was likely responsible for the effect ( Fig. 10c and Supplementary Fig. 10 ). 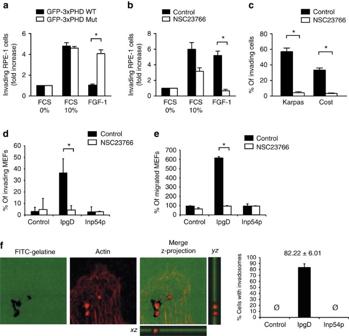Figure 10: PtdIns5P is required for invasion of dense Matrigel and invadosome formation. (a) Invasiveness of transduced RPE-1 cells into 3D-Matrigel toward a FBS gradient or FGF-1 was examined using transwell chambers. The number of cells penetrating the Matrigel was expressed as a fold increase compared with the experiment without serum gradient. Data are shown as mean±s.e.m. (n=3; *P<0.05 using non-parametric one way ANOVA (Kruskal–Wallis) with Dunn’s post test) (b) Same experiment as in (a) except that RPE-1 were treated overnight with NSC23766 (100 μM). Data are shown as mean±s.e.m. (n=3; *P<0.05 using non-parametric one way ANOVA (Kruskal–Wallis) with Dunn’s post test). (c) Karpas 299 or Cost cells were treated overnight with NSC23766 (40 μM) before CMTMR staining. Invasiveness towards an FBS and 1 μg ml−1SDF1α gradient was examined. The number of cells penetrating the Matrigel to depths of 20 μm and greater was expressed as a percentage of the total cell number within the gel. Data are shown as mean±s.e.m. (n=3; *P<0.05 using non-parametric one way ANOVA (Kruskal–Wallis) with Dunn’s post test). (d) IpgD or Inp54p expression was induced in MEF Tet-Off cells before serum starvation. Then, invasiveness into 3D-Matrigel ±NSC23766 (100 μM) towards an FBS gradient was examined. Data are shown as mean±s.e.m. (n=3; *P<0.05 using non-parametric one way ANOVA (Kruskal–Wallis) with Dunn’s post test). (e) Serum-starved control, IpgD or Inp54p-expressing MEFs were seeded into transwell chambers. Migration toward a gradient of FBS was allowed for 6 h ±NSC23766 100 μM and the percentages of migrated cells were determined. Data are shown as mean±s.e.m. (n=3 experiments; *P<0.05 using non-parametric one-way ANOVA (Kruskal–Wallis) with Dunn’s post test). (f) MEF-IpgD were cultured on FITC-gelatin-coated coverslips for 24 h. Degradation areas were visualized as dark holes.zprojections show that actin cores are present within the degraded gelatin. The percentage of cells that presented at least one area of gelatin degradation was determined. Data are shown as mean±s.e.m. (n=3). Figure 10: PtdIns5P is required for invasion of dense Matrigel and invadosome formation. ( a ) Invasiveness of transduced RPE-1 cells into 3D-Matrigel toward a FBS gradient or FGF-1 was examined using transwell chambers. The number of cells penetrating the Matrigel was expressed as a fold increase compared with the experiment without serum gradient. Data are shown as mean±s.e.m. ( n =3; * P< 0.05 using non-parametric one way ANOVA (Kruskal–Wallis) with Dunn’s post test) ( b ) Same experiment as in ( a ) except that RPE-1 were treated overnight with NSC23766 (100 μM). Data are shown as mean±s.e.m. ( n =3; * P< 0.05 using non-parametric one way ANOVA (Kruskal–Wallis) with Dunn’s post test). ( c ) Karpas 299 or Cost cells were treated overnight with NSC23766 (40 μM) before CMTMR staining. Invasiveness towards an FBS and 1 μg ml −1 SDF1α gradient was examined. The number of cells penetrating the Matrigel to depths of 20 μm and greater was expressed as a percentage of the total cell number within the gel. Data are shown as mean±s.e.m. ( n =3; * P< 0.05 using non-parametric one way ANOVA (Kruskal–Wallis) with Dunn’s post test). ( d ) IpgD or Inp54p expression was induced in MEF Tet-Off cells before serum starvation. Then, invasiveness into 3D-Matrigel ±NSC23766 (100 μM) towards an FBS gradient was examined. Data are shown as mean±s.e.m. ( n =3; * P< 0.05 using non-parametric one way ANOVA (Kruskal–Wallis) with Dunn’s post test). ( e ) Serum-starved control, IpgD or Inp54p-expressing MEFs were seeded into transwell chambers. Migration toward a gradient of FBS was allowed for 6 h ±NSC23766 100 μM and the percentages of migrated cells were determined. Data are shown as mean±s.e.m. ( n =3 experiments; * P< 0.05 using non-parametric one-way ANOVA (Kruskal–Wallis) with Dunn’s post test). ( f ) MEF-IpgD were cultured on FITC-gelatin-coated coverslips for 24 h. Degradation areas were visualized as dark holes. z projections show that actin cores are present within the degraded gelatin. The percentage of cells that presented at least one area of gelatin degradation was determined. Data are shown as mean±s.e.m. ( n =3). Full size image IpgD expression and subsequent PtdIns5P elevation were capable of switching the phenotype of MEFs to highly motile and invasive cells, which correlated with the observed increase in membrane and actin dynamics, while control MEFs or MEF-Inp54p showed no 2D nor 3D motility ( Fig. 10d,e and Supplementary Fig. 11a ). In this model, inhibition of Tiam1/Rac1 by NSC23766 blocked both migration and invasion as observed for RPE-1 cells challenged with FGF-1 ( Fig. 10b–d ). We then assessed in situ the proteolytic activity of MEF-IpgD using fluorescent-matrix degradation assays. After 48 h, ~\n80% of cells displayed degradation areas ( Fig. 10f ). Invadopodia/invadosomes are small needle-like membrane projections located at sites of major structural dynamics where proteolytic degradation occurs, at the ventral side of cells in 2D and in the direction of the gradient in 3D [46] , [47] . By immunofluorescence, invadosomes appear as patched structures enriched in proteins that regulate cytoskeleton and membrane remodelling, cell–ECM adhesion and matrix degradation [47] . Confocal sections followed by orthogonal plotting of the images ( z projection) demonstrated that the digested zones contained cores of F-actin, a trademark of functional invadosomes ( Fig. 10f ). The above observations demonstrated for the first time that PtdIns5P orchestrates invasion through activation of Tiam1 and Rho GTPases to restrict actin dynamics and allow matrix digestion. In this paper, we unravelled a new role for non-nuclear PtdIns5P in cell invasion where it increases actin and membrane dynamics through activation of the Tiam1/Rac1 module. We studied three different pathophysiological situations, stimulation of RPE-1 cells by FGF-1, ectopic expression of the bacterial IpgD phosphatase and transformation by the NPM-ALK oncogene, and showed that they all relied on this pathway to elicit 3D migration. We used the Raichu probe to assess active Rac1 in cells. It is known that this probe does not bind RhoGDI, suggesting it might not behave in the same manner as endogenous Rac1. However, Raichu-Rac1 has been shown to interact with other important regulators of GTPases such as GAPs and GEFs, among which is Tiam1, to regulate its local activity [48] . Confocal microscopy allowed us to detect FRET at sites of endogenous Rac1 localization, ruffles and vesicles. Recently, it was demonstrated that recruitment of Tiam1 and Rac1 to early endosomes upon endocytosis or activation of receptor tyrosine kinases (RTKs) was required for the spatial partitioning of active Rac to zones where protrusive activity led to motility [42] , [49] . However, the molecular mechanism for this recruitment was not studied. Our findings indicate that PtdIns5P might be the missing link between trafficking and actin/membrane dynamics. We found a direct binding between PtdIns5P and the Tiam1 PHc domain that localized it to early endosomes and led to chemotaxis. These findings shed new light on the complex relationship between PIs and GEFs for Rho GTPases [50] . PIs interact with GEFs through the PH domain associated to the DH domain responsible for their exchange activity. GEFs are then localized at PI-enriched membrane regions to activate their target GTPases and engage downstream signalling for an accurate response to the initial insult. However, most PH domains found in the DH-PH tandem bind poly-PIs (PtdIns(4,5)P 2 and PtdIns(3,4,5)P 3 ) with low affinity and often require protein adaptors for efficient membrane association. A careful survey of the literature highlights the fact that no systematic studies have been undertaken to clearly assess the specificity of GEF PH domains [50] . By adapting a method whereby Rac1 can be anchored to liposomes bearing different PtdInsP, we could demonstrate that PtdIns5P binding by Tiam1 DH-PHc potentiates its intrinsic GEF function. GEF activation is in part due to an improved probability for the formation of complexes containing all three partners (Tiam1 DH-PHc, Rac1 and PtdIns5P). However, since GEF DH-PH domains have weak activity in solution, it also can be postulated that binding to PtdIns5P-bearing liposomes favours a more active conformation of the DH-PH towards interaction and exchange on Rac1 (ref. 38 ). Our method represents a significant improvement since previous studies failed to demonstrate any effect on GEF activity via Tiam1 DH-PHc interaction with PtdIns3P in solution [36] . We confirmed that PtdIns3P bound Tiam1 PHc, albeit with a lower affinity than PtdIns5P. In agreement, we could measure a weak activation by PtdIns3P-bearing liposomes, demonstrating that both PIs could activate Tiam1 in vitro . This observation has an important impact on cells, since we have previously demonstrated that PtdIns5P accumulation on early endosomes, known to be enriched in PtdIns3P, induced trafficking modifications. Indeed, Palamidessi et al. [42] and Joffre et al. [49] demonstrated that the activation of, respectively, Tiam1/Rac1 and Rac1 and oncogenic mutants of the Met receptor on early endosomes was instrumental to directed motility. In HeLa and BHK cells, PtdIns5P endosome enrichment led to stabilization and sustained activation of EGFR by blocking its degradation and favoring recycling [10] . Endocytosis and trafficking have long been regarded merely as means of attenuating cell activation through degradative pathways. The concept of ‘signalling endosomes’, which stems from the observation that signalling persists along the endocytic route, shed new light on how signalling pathways are regulated [51] . Our findings demonstrate that the assumption that endosomal PtdIns3P accounted for those effects is not totally accurate and identify PtdIns5P as an important component of endosome-associated signalling. Since IpgD does not lead to modification of total nor endosomal PtdIns3P levels, our study indicates that PtdIns5P is the main PI that recruits Tiam1 to early endosomes when high levels of PtdIns5P are present. In this line of thought, localization of PtdIns3P and PtdIns5P in MEF-IpgD demonstrated that they colocalized on endomembranes. However, only PtdIns5P was enriched at the plasma membrane and in ruffles ( Supplementary Fig. 9 ). Therefore, it is possible that under basal conditions, when PtdIns3P and PtdIns5P are present in comparable amounts, they could cooperate to achieve balance between degradation and recycling of cargo during steady state trafficking. In FGF-1 signalling and NPM-ALK lymphomas, PIKfyve, either alone or in coordination with MTMR3, has been demonstrated to modulate the levels of PtdIns3P, PtdIns(3,5)P 2 and PtdIns5P (refs 15 , 21 , 28 ). However, in all cases, sequestration of PtdIns5P by the GFP-3xPHD probe and complementation of PIKfyve knock down by synthetic PtdIns5P or IpgD transfection demonstrated that, indeed, PtdIns5P was the important PI for effects on actin and migration. Interestingly, our study opens a new field of investigation on GEFs as interacting partners and effectors of PtdIns5P, likely accounting for some of the non-nuclear PtdIns5P functions. Moreover, Miroshnychenko et al. [52] reported that the PH domain of BCR also showed affinity for PtdIns5P, but they did not investigate it further. Additional studies are required to elucidate the existence of PtdIns5P-responsive subfamilies of Rho GTPases and GEFs. Our findings demonstrate that activation of Tiam1/Rac1 by PtdIns5P is a potent signal that can reprogram non-migrating cells to engage in both 2D- and 3D-directed migration. Indeed, MEFs expressing high levels of PtdIns5P undergo a phenotypical modification reminiscent of cancer-associated fibroblasts and fibroblasts activation during wound-healing processes [53] , where they become highly invasive by increased motility and through secretion of MMPs. Circular dorsal ruffles, also called ‘waves’, share regulatory circuitry similar to invadosomes, which drive motility in 3D matrices [44] . Cdc42 is a central element of invadosome structure and function [54] . Upon PtdIns5P increase, Cdc42 is activated and regulates cortical actin, which might cooperate with Rac1 to generate invadosomes. Accordingly, this work and our previous studies demonstrated that Rac1 was required to trigger matrix digestion [18] , [19] , [20] . The discovery that PtdIns5P is a central regulator of ECM remodelling, actin and membranes dynamics, which are prerequisites for 3D migration, broadens our view of how this phenomenon is regulated. In conclusion, the sum of our work demonstrates that PtdIns5P is an important mediator of signalling, leading to invasion/3D migration in response to different extracellular or oncogenic cues. The outcome of PtdIns5P elevation and of Tiam1/Rac1 activation elicited by either RTK activation (FGF-1 or insulin [17] ), bacterial infection or tumorigenesis can be either beneficial, in the case where physiological development requires accurate cell motility, or detrimental, when exploited in pathologies such as cancer, diabetes or bacterial infection. Therefore, this work points to PtdIns5P as a crucial mediator involved in determining cellular fate by acting at the crossroads of cellular processes such as trafficking, motility and response to growth factors that have high pathophysiological relevance. Targeting enzymes involved in its metabolism represent therapeutic targets worth exploring for a wide array of diseases. Reagents and antibodies NSC23766 was from Calbiochem, secramine A and YM201636 were generous gifts from T. Kirchhausen (Harvard Medical School, USA) and P. Parker (London Research Institute, UK) respectively. Fibronectin micropatterned chips were from CYTOO. FGF-1 was from Peprotech. GST-Rac1-G15A and GST-Cdc42-G15A beads were from Cell Biolabs or were purified as described [55] . Antibodies used in this study are listed in Supplementary Table 1 . Horseradish peroxidase-conjugated goat anti-mouse and anti-rabbit immunoglobulin antisera were from Promega. AlexaFluor-labelled secondary antibodies were from Life Technologies. Synthetic lipids were from Avanti Polar Lipids and Echelon. shRNA expression vectors directed against PIKfyve were from Sigma-Aldrich: TRCN0000150008 (sh1: 5′-CCTTGGATTGTAACAATGG-3′), TRCN0000147783 (sh2: 5′-GCCAAGTCTATTCAAGTCT-3′). Mission turbo GFP was used as a control. Cell culture, plasmids and transfection Tet-Off MEF cells were grown in DMEM supplemented with 10% FBS, 100 U ml −1 penicillin, 100 μg ml −1 streptomycin and 500 μg ml −1 G418 (Life Technologies). Wild-type and Tiam1 −/− knockout MEFs, cultured in DMEM supplemented with 10% FBS and 50 μM ß-mercaptoethanol, were provided by J. Collard and A. Malliri (Netherlands Cancer Institute, the Netherlands and University of Manchester, UK, respectively). The ALCL cell lines Cost and Karpas 299 (harbouring the t(2,5)(p23;q35) translocation and expressing NPM-ALK) were cultured in IMDM (Life Technologies) supplemented with 15% FBS. Cost ALCL cell line [56] was obtained from F. Meggetto (INSERM U1037, France). Karpas 299 ALCL cells were obtained from DSMZ (German Collection of Microorganisms and Cell Culture, Germany). RPE-1 cells were provided by B. Goud (Curie Institute, France). Cell lines were checked twice a month for Mycoplasma (Lonza). DNA transfections were performed using Lipofectamine with Plus Reagent (Life Technologies) or X-tremeGENE 9 (Roche) according to the manufacturer’s instructions. For treatment with short-chain lipids, C4-PtdIns4P and C4-PtdIns5P (Echelon Biosciences Inc.) were resuspended in water and used at 15 μM for the indicated time on serum-starved MEF cells, except where stated otherwise. The following plasmids were used: pRK5-Myc-IpgD, pCDNA3-EGFP-Lyn-Inp54p vector (gift from T. Meyer, Stanford University, USA), pRaichu-Rac1, pRaichu-Cdc42, pEGFP-actin (gift from B. Geny, Pasteur Institute, France), pEGFP-N3-NPM-ALK (gift from M. Fawal, Spanish National Cancer Research Center, Spain), pcDNA3-HA-Tiam1 (gift from A. Malliri, University of Manchester, UK), pGEX-2TK-DH-PH-Tiam1 WT, mutant L2, mutant L1/L2, (myc-tagged) FL PH*L1/L2 Tiam-1 were a gift from M.A. Lemmon (University of Pennsylvania, USA). WT Rac-His was obtained by site-directed mutagenesis using the pET28a-Rac1-Q61L vector as a template (gift from J.R. Peterson, Fox Chase Cancer Center, USA). pRaichu-1026x bearing the CAAX box of Rac1 before CFP was a gift from Dr Matsuda (Osaka University, Japan). pGEX-4T1-PHn Tiam1 was obtained by sub-cloning using pcDNA3-HA-Tiam1 as a template. Establishment of MEFs inducible cell lines EGFP-IpgD, EGFP-Inp54p or EGFP-IpgD-C438S were subcloned into the pTRE2-hyg-Myc expression vectors (Clontech) by standard techniques. A total of 1 × 10 6 MEF Tet-Off cells (Clontech) expressing the tetracycline-controlled transactivator were plated in 100 mm dishes and transfected with 2 μg of pTRE2-hyg-Myc-EGFP-IpgD, pTRE2-hyg-Myc-EGFP-Inp54p or pTRE2-hyg-Myc-EGFP-IpgD-C438S using Lipofectamine with Plus Reagent (Life Technologies) and 2 μg ml −1 of doxycyclin (Sigma-Aldrich) was added to avoid any protein expression during the selection process. Forty-eight hous after transfection, 400 μg ml −1 of hygromycin (Sigma-Aldrich) was added. Transformants were selected and single cells cloned using the limiting dilution method. To test for induced expression, doxycyclin was removed from the medium and EGFP-positive clones were selected and analysed by western blot for expression of Myc-EGFP-IpgD, Myc-EGFP-Inp54p or Myc-EGFP-IpgD-C438S. Lentivirus production and transduction EGFP-3xPHD WT and EGFP-3xPHDmut (cysteine mutant)-encoding sequences were subcloned from the pEGFP-C1 plasmids [8] into the pTRIP-IRES lentiviral vector plasmid [57] . Vector particles were produced as previously described [57] . Cost and Karpas 299 cells were transduced by incubation with lentiviral particles at an MOI of 1. Cells were washed 24 h later and after an additional 48 h, EGFP-positive cells were sorted by flow cytometry on a BD FACSAria Sorp (BD Biosciences). RPE-1 cells were transduced by incubation with lentiviral particles at an MOI of 1 for 3 days. Transduction efficiency was checked by fluorescence microscopy and reached almost 100%. Cost and Karpas cells were transduced by incubation with lentiviral particles at an MOI of 1 for 3 days and selected using 2 μg ml −1 puromycin. Immunoprecipitation and western blotting Total cellular proteins were extracted with 50 mM Tris-base (pH 8), 150 mM NaCl, 5 mM EGTA, 1% Nonidet P-40, 1 mM PMSF, 50 mM NaF, 1 mM Na 3 VO 4 , 10 mg ml −1 leupeptin and 2 mg ml −1 aprotinin. For cell fractionation, cells were scraped in detergent-free lysis buffer as described above. Homogenates were centrifuged for 10 min at 1,000 g . The post-nuclear supernatant was then centrifuged for 30 min at 100,000 g . The supernatant (HSS) was collected and the pellet resuspended in lysis buffer supplemented with 1% TritonX-100 and 0.5% sodium deoxycholate to obtain the membrane fractions (HSP). For immunoprecipitations, clarified homogenates were incubated overnight at 4 °C with the antibodies and a mix of protein A/G sepharose beads. After washes, proteins were eluted with Laemmli buffer and analysed by SDS-PAGE followed by western blotting on Immobilon-P membranes (Millipore) with appropriate antibodies. Immunoreactive bands were detected by chemiluminescence using either medical X-ray film (Kodak) or chemidoc (Bio-Rad Laboratories) with the SuperSignal detection system (Pierce). Quantification was done using ImageJ or Chemidoc Image lab (Biorad laboratories). Larger images of immunoblots shown in the main article are included in Supplementary Fig. 12,13 and 14 . GTPase pull-downs and GEF trapping The amounts of GTP-bound active Rac1, Cdc42 or RhoA and active Tiam1 were determined by pull-downs as previously described [55] , [58] . Briefly, cells were lysed in ice-cold lysis buffer (50 mM Tris-base (pH 7.4), 500 mM NaCl, 10 mM MgCl 2 , 2.5 mM EGTA, 1% Triton X-100, 0.5% sodium deoxycholate, 0.1% SDS, 1 mM PMSF, 50 mM NaF, 1 mM Na 3 VO 4 , 10 μg ml −1 leupeptin and 2 μg ml −1 aprotinin) and clarified lysates were incubated with 20 μg GST-PBD (PAK1 Binding Domain for Rac1 and Cdc42), GST-RBD (Rhotekin Binding Domain for RhoA) or GST-Rac1G15A (for GEF trapping assays) beads at 4 °C for 60 min. After washes, bound proteins were eluted with Laemmli buffer and analysed by SDS–PAGE followed by western blotting. Microscopy FRET efficiency was represented as the color-coded ratio image of YFP/CFP after background subtraction using MetaMorph (Universal Imaging). Some experiments were conducted using a wide-field microscope (Axiovert 200, Carl Zeiss) with a × 40 oil immersion lens (Carl Zeiss). MetaMorph was used for acquisition with a CoolSNAP HQ camera (Roper Scientific). The filters used for the dual-emission ratio imaging were a 455DRLP dichroic mirror and two emission filters, 470AF40 for CFP and 535BP35 for YFP (Chroma Technology Corp). Cells were illuminated with a 75 W xenon lamp through a 20 nm bandwidth monochromator Optoscan (CAIRN Research Limited) at 435 nm for CFP excitation and 500 nm for YFP excitation. The exposure time was 0.5 s with 3 × 3 binning, every minute. After the first acquisition, 0.5 μM PtdInsPs were added to the cells. Other FRET experiments were performed with a confocal microscope LSM 780 piloted by the Zen software, using a × 40 Plan-Apochromat water immersion lens (Carl Zeiss). Images were acquired with a pinhole diameter of 149 μm. For immunofluorescence, cells were fixed/permeabilized for 20 min in 3.7% formaldehyde with 0.05% TritonX100 and saturated in 1% fatty acid free BSA/PBS. Incubation with antibodies or the GST-2xPHD probe (40 μg ml −1 in 1% BSA/PBS) was performed for 30 min at room temperature. After incubation with fluorescent secondary antibodies or AlexaFluor-labelled phalloidin (Molecular Probes), cells were washed with PBS and mounted with Mowiol. Confocal imaging was performed using a LSM 710 or 780 microscope, piloted by Zen software, with a × 63 Plan-Neofluar objective (Carl Zeiss). Profiling of fluorescence intensity was done with ImageJ. Phospholipid extraction and analysis Phospholipids were extracted and analysed by high-performance liquid chromatography (HPLC) after metabolic labelling with [ 32 P]orthophosphate (200 μCi ml −1 ; Perkin Elmer), except for PtdIns3P and PtdIns5P that were quantified by mass assay as described [13] , [14] , [24] . Briefly, total lipid extraction was performed according to the Bligh and Dyer procedure [59] . PtdInsP were then purified by thin layer chromatography. Lipid kinase assays were performed using recombinant PIKfyve (for PtdIns3P) and PI5P 4-kinase IIα (for PtdIns5P) and [γ- 32 P]ATP (Perkin Elmer). The radioactive biphosphates generated (proportional to the PtdIns3P or PtdIns5P present in the sample) were extracted and analysed by HPLC. Lipid–protein overlay assay (fat blots) Recombinant GST-tagged proteins were expressed in E.coli strain BL21(DE3) and purified by affinity chromatography using glutathione Sepharose 4B beads according to the manufacturer’s instructions ( GE Healthcare). PIP-Strips (Echelon Biosciences Inc) and in-house membranes were used as previously described [60] . Membranes were blocked in TBS or PBS containing 3 mg ml −1 FA-free BSA and 0.1% Tween 20. Incubations were done with 0.5 μg ml −1 of purified protein in blocking buffer. After washes, binding of the domains to the PIs was detected by anti-GST western blotting. Liposome-binding assays The liposome-binding assays were performed essentially as previously described [61] . Briefly, liposomes containing PC:PE (50:50) or PC:PE:PtdInsP(n) (45:45:10) were prepared by mixing chloroform stocks, drying and resuspending using a bath sonicator in 10 mM HEPES (pH 7.7), 100 mM NaCl, 200 mM sucrose and 5 mM EGTA. Liposome sedimentation assays were conducted using 300 μM liposomes and 2 μg of GST fusion proteins. All centrifugation steps were done at 16,000 g and 4 °C. Supernatant and pellet fractions were analysed by SDS–PAGE and silver staining. Binding of Rac-His to liposomes Liposomes containing PC:PE:PE-fluorescein:DGS-NTA(Ni) (67:28:2:3) were prepared by mixing chloroform/methanol stocks, drying and resuspending in 50 mM HEPES (pH 7.5), 100 mM NaCl, 200 mM sucrose and 5 mM EGTA. After vortexing and 10 min equilibration at room temperature, the suspension was subjected to five freeze/thaw cycles using liquid nitrogen and extruded 19 times through 0.1 μm polycarbonate filter using a hand extruder (Avanti Polar Lipids). Liposomes were kept at 4 °C and used within 4 days of their preparation. Increasing concentrations of Rac-His were incubated with 300 μM liposomes for 20 min at room temperature in 50 mM HEPES (pH 7.5), 120 mM Potassium acetate, 1 mM MgCl2 and 1 mM DTT. Liposomes were then pelleted by centrifugation (1 h, 16,000 g , 20 °C) and the fluorescent liposome pellet was visualized using a UV lamp. Supernatant and pellet fractions were analysed by SDS–PAGE and Coomassie staining (Imperial protein stain, Thermo scientific). Exchange factor activity Liposomes were prepared as described in the Methods for ‘Binding of Rac-His to liposomes’ but without sucrose. Liposome compositions were PC:PE:DGS-NTA(Ni) (67:30:3) and PC:PE:DGS-NTA(Ni):PtdInsP (61:30:3:6). All incubations were done in 96-well black microplates in a final volume of 100 μl. Rac-His (loaded with bodipy FL GDP) (1 μM) was incubated with liposomes (300 μM) for 10 min in 50 mM Tris (pH 7.5), 100 mM NaCl, 10 mM MgCl 2 . Then, 100 nM Tiam1 DH-PHc (GST-tag was cleaved with thrombin) was added for 10 additional minutes. Reaction was started by adding 400 μM GTP. Activation of Rac1 was monitored by fluorescence of bodipy (488/535 nm). Fluorescence intensity was recorded every 15 s for 40 min using a Varioskan flash spectrofluorometer (Thermo scientific). All measurements were performed at 30 °C. Migration and invasion assays For transwell experiments, cells were processed as described [18] . Briefly, cells were seeded in 24-well plates in transwell chambers (BD Biosciences). Migration proceeded for 6 h toward a gradient of FBS from the upper chamber of the transwell insert (without FBS) to the lower chamber (with 10% FBS), where cells were scored. Matrigel matrix (BD Biosciences) invasion assay was performed on 20,000 serum-starved cells for 6 h and labelled for 90 min with 0.5 μM CellTracker Orange CMTMR (Life Technologies). After washes, cells were seeded in labtek chambers and overlaid with Matrigel at 5 mg ml −1 , ±100 μM NSC23766 (40 μm for Cost and Karpas 299). After 90 min at 37 °C, medium containing 10% FBS was added (15% FBS containing 1 μg/ml SDF1α for Cost and Karpas 299 cells). Optical z sections were taken every 2.5 μm starting from the base and extending 100 μm into the Matrigel. A representative image is shown in Supplementary Fig. 10 . To quantify invasion, CMTMR fluorescent cells in the sections above 20 μm were added and then divided by the sum of cells in all z sections. Quantification was performed using Imaris 6.4.2 software (Bitplane). For transwell experiments, cells were processed as described [18] . Briefly, cells were seeded in 24-well plates in transwell chambers (BD Biosciences). Migration proceeded for 6 h toward a gradient of FBS from the upper chamber of the transwell insert (without FBS) to the lower chamber (with 10% FBS), where cells were scored, either after staining with crystal violet or after fixation, permeabilization and DAPI staining. Representative images are shown in Supplementary Fig. 11 . ECM degradation assays Cells were seeded on FITC-gelatin-coated coverslips as described previously [62] . For colocalization experiments, cells were fixed, stained and analysed as described above using a LSM 780 confocal microscope. To quantify ECM degradation, we determined the percentage of cells that presented areas of degradation relative to the total number of cells in each condition. Duolink in situ proximity ligation assay Cells grown on coverslips were fixed in 3.7% formaldehyde and permeabilized with 0.2% Triton X-100. Coverslips were then incubated with primary antibodies for 1 h, except in the case of PtdIns5P detection where the coverslips were incubated with GST-2xPHD probe before incubation with an anti-GST antibody as primary. Hybridization, ligation, amplification and detection were realized according to the manufacturer’s instructions (Olink Bioscience). In brief, secondary antibodies were incubated in a humidity chamber for 1 h at 37 °C. Ligation was performed with a ligase-containing ligation solution for 30 min at 37 °C. Then, the amplification step was performed with a polymerase-containing amplification solution for 1 h and 40 min at 37 °C. Coverslips were analysed by confocal imaging using a LSM 780 microscope, piloted by the Zen software, with a × 63 Plan-NEOFLUAR objective (Carl Zeiss). Duolink fluorescent dots were counted using the ‘analyse particles functions’ of the Fiji software. Statistical analysis Data are representative of three to five independent experiments and provided as mean±s.e.m. Statistical analyses were carried out by either non-parametric t -test, non-parametric one-way ANOVA (Kruskal–Wallis) with Dunn’s post test or one sample t -test (for the deviation from mean value in a control group) using GraphPad PRISM 4.0 software (GraphPad Software Inc., La Jolla, CA, USA). Significance was accepted at * P< 0.05. The number of cells analysed in the various experiments presented herein can be found in Supplementary Table 2 . How to cite this article: Viaud, J. et al. Phosphatidylinositol 5-phosphate regulates invasion through binding and activation of Tiam1. Nat. Commun. 5:4080 doi: 10.1038/ncomms5080 (2014).